Pharmacological repression of PPARγ promotes osteogenesis The nuclear receptor peroxisome proliferator-activated receptor gamma (PPARγ) is the master regulator of adipogenesis and the pharmacological target of the thiazolidinedione (TZD) class of insulin sensitizers. Activation of PPARγ by TZDs promotes adipogenesis at the expense of osteoblast formation, contributing to their associated adverse effects on bone. Recently, we reported the development of PPARγ antagonist SR1664, designed to block the obesity-induced phosphorylation of serine 273 (S273) in the absence of classical agonism, to derive insulin-sensitizing efficacy with improved therapeutic index. Here we identify the structural mechanism by which SR1664 actively antagonizes PPARγ, and extend these findings to develop the inverse agonist SR2595. Treatment of isolated bone marrow-derived mesenchymal stem cells with SR2595 promotes induction of osteogenic differentiation. Together these results identify the structural determinants of ligand-mediated PPARγ repression, and suggest a therapeutic approach to promote bone formation. Central to the lineage commitment of multipotent mesenchymal stem cells (MSCs) is the nuclear receptor peroxisome proliferator-activated receptor gamma (PPARγ), the master regulator of adipogenesis and the pharmacological target of the thiazolidinedione (TZD) class of insulin sensitizers [1] . Activation of PPARγ by the TZDs promotes adipocyte differentiation at the expense of osteoblast formation, contributing to their associated adverse effects on bone [2] . To address these concerns, a novel class of partial agonist selective PPARγ modulators (SPPARγMs) were developed that display reduced expression of PPARγ-target genes, while maintaining potent insulin-sensitizing efficacy similar to that of full agonist TZDs [3] . SPPARγMs demonstrate the ability to decouple PPARγ activation and insulin-sensitizing efficacy, while showing improvement for several TZD-associated adverse effects in animal models of diabetes [4] . Recently, it was demonstrated that the obesity-induced phosphorylation of PPARγ at Serine 273 (pS273) leads to repression of a subset of the receptors’ target genes associated with insulin resistance [5] . The efficacy of SPPARγMs and TZDs was shown to correlate with their ability to block pS273, leading to normalization of the dysregulated PPARγ-target gene set. On the basis of these findings, an alternative class of high-affinity functional SPPARγMs was developed that effectively block pS273, while avoiding classical activation function 2 (AF2)-driven receptor activation [6] . SR1664 is a representative compound from this class of PPARγ modulators that was shown in vivo to be similarly efficacious at insulin sensitizing as rosiglitazone, with further improvements on adverse effect markers relative to SPPARγMs. Here we report the structural mechanism by which SR1664 actively antagonizes PPARγ through an AF2-mediated clash, and extend these findings to enable the structure guided design of the inverse agonist SR2595. Consistent with the desirable bone phenotype observed in PPARγ-deficient animal models [7] , we demonstrate that pharmacological repression of PPARγ promotes osteogenesis in cultured MSCs. SR2595 has sufficient pharmacokinetics to support in vivo studies and demonstrates no negative effects on metabolic parameters in 21-day treated C57BL/6 mice. Together these results demonstrate the effect of pharmacological PPARγ repression on MSC lineage commitment, and suggest a therapeutic approach to promote bone formation devoid of adverse effect on metabolic parameters. Structural mechanism of PPARγ active antagonism Efforts to develop structure activity relationship (SAR) around the antagonist SR1664 began with an unexpected observation that its R -enantiomer SR1663 ( Fig. 1a ) is an agonist that potently activates PPARγ as defined in a co-transfection promoter:reporter assay ( Fig. 1b ). To elucidate the structural mechanism driving this stereo-specific functional divergence, co-crystal structures of the PPARγ ligand-binding domain (LBD) in complex with SR1664 and SR1663 were both solved to a resolution of 2.3 Å ( Fig. 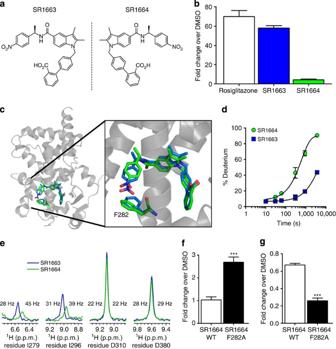Figure 1: Structure activity relationship around enantiomers SR1663 and SR1664. (a) Chemical structures of SR1664 andR-enantiomer SR1663. (b) Transcriptional activity of a PPARγ-Gal4:UAS-Luciferase promoter–reporter assay in HEK293T cells with 1 μM ligand. (c) Alignment of PPARγ:SR1663 (blue) and PPARγ:SR1664 (green) co-crystal structures. Zoomed panel highlights stereo-specific interaction with residue F282. (d) HDX buildup curves of PPARγ LBD helix 3 peptide (IRIFQGCQ) containing F282 in the presence of SR1663 and SR1664. (e) Extracted one-dimensional plots from two-dimensional [1H,15N]-TROSY-HSQC NMR data for PPARγ LBD in the presence of SR1663 or SR1664; half-height resonance line widths are indicated. (f) Transcriptional activity of wild type versus F282A PPARγ in PPARγ:PPRE-Luciferase promoter–reporter assay with 1 μM SR1664 in HEK293T cells. (g) Wild type versus F282A PPARγ:NCoR NR Box 1 peptide affinity with 1 μM SR1664 in TR-FRET assay. Error bars, s.e.m; one-way analysis of variance, Dunnett’spost hoctest *P<0.05, **P<0.01, ***P<0.001. 1c ; Table 1 ). Structural alignment revealed no significant differences in the overall global conformation of the LBD (RMSD C α =1.14 Å), consistent with previously reported PPARγ co-crystal structures [8] . The ligands partially overlap with their biphenyl and indole moieties closely aligned. However, the positioning of the nitro substituent diverges with SR1663 making a favourable pi stacking interaction with phenylalanine 282 (F282 PPARγ1 numbering; PPARγ2 F310) on helix 3, while SR1664 exhibits a steric clash with F282 ( Fig. 1c ). SR1664 binding to the PPARγ LBD resulted in an increased rate of hydrogen/deuterium exchange (HDX) for helix 3 relative to that observed on binding SR1663, consistent with disruption of intra-helix hydrogen bonding due to the steric clash with F282 ( Fig. 1d ). Increased NMR resonance line widths indicate SR1664 increases μs–ms dynamics relative to SR1663, both near the clash site (I279) and distal on helix 3 (I296) ( Fig. 1e ). Mutagenesis of F282 to alanine (F282A) altered the pharmacology of SR1664 on PPARγ activity, acting as an agonist of the mutant receptor in a transcriptional activity assay ( Fig. 1f ), and differentially displacing nuclear receptor co-repressor 1 ( Fig. 1g ). Together these results suggest that SR1664 actively antagonizes PPARγ through a stereo-specific AF2-mediated, F282-dependent clash, and that stereospecificity confers antagonism within the biaryl indole scaffold. Figure 1: Structure activity relationship around enantiomers SR1663 and SR1664. ( a ) Chemical structures of SR1664 and R -enantiomer SR1663. ( b ) Transcriptional activity of a PPARγ-Gal4:UAS-Luciferase promoter–reporter assay in HEK293T cells with 1 μM ligand. ( c ) Alignment of PPARγ:SR1663 (blue) and PPARγ:SR1664 (green) co-crystal structures. Zoomed panel highlights stereo-specific interaction with residue F282. ( d ) HDX buildup curves of PPARγ LBD helix 3 peptide ( IRI F QGCQ ) containing F282 in the presence of SR1663 and SR1664. ( e ) Extracted one-dimensional plots from two-dimensional [ 1 H, 15 N]-TROSY-HSQC NMR data for PPARγ LBD in the presence of SR1663 or SR1664; half-height resonance line widths are indicated. ( f ) Transcriptional activity of wild type versus F282A PPARγ in PPARγ:PPRE-Luciferase promoter–reporter assay with 1 μM SR1664 in HEK293T cells. ( g ) Wild type versus F282A PPARγ:NCoR NR Box 1 peptide affinity with 1 μM SR1664 in TR-FRET assay. Error bars, s.e.m; one-way analysis of variance, Dunnett’s post hoc test * P <0.05, ** P <0.01, *** P <0.001. Full size image Table 1 Data collection and refinement statistics. Full size table Structure guided design of PPARγ inverse agonist SR2595 On the basis of this emerging SAR, it was hypothesized that furthering the AF2 clash observed with SR1664, through addition of a bulkier substituent could result in repression of basal receptor activity [9] . Indeed, SR2595, substitution of t-butyl for nitro at the para position of SR1664, repressed transactivation in a promoter:reporter assay ( Fig. 2a,b ; binding affinity for analogues are provided in Supplementary Table 1 ) and expression of the adipogenic marker fatty acid-binding protein 4 ( FABP4 ) in differentiating murine preadipocytes below basal levels ( Fig. 2c ). This inverse agonist SAR was conserved across several optimized analogues of SR2595 including SR10221 ( Fig. 2a–c ; Supplementary Fig. 1a ). Similar to that observed with the antagonist SR1664, mutagenesis of F282A altered the pharmacology of SR2595 to act as an agonist in transactivation, and on displacement of nuclear receptor co-repressor 1 ( Supplementary Fig. 1b,c ). HDX kinetics of the PPARγ LBD demonstrated a strong correlation between transactivation and ligand-induced protection of helix 12, a surface of the receptor critical for cofactor interaction and ligand-dependent receptor transactivation ( Fig. 2d ). NMR resonances for residues proximal to helix 12 (L465 and H466) were observed only for agonists rosiglitazone and SR1663, indicative of multiple conformational sampling by these residues with PPARγ bound to either antagonist SR1664 or inverse agonists SR2595 and SR10221 ( Fig. 2e ). These findings demonstrate the structural determinants guiding the design of PPARγ inverse agonist SR2595, and provide a pharmacological approach to repress PPARγ activity and block basal adipogenesis. 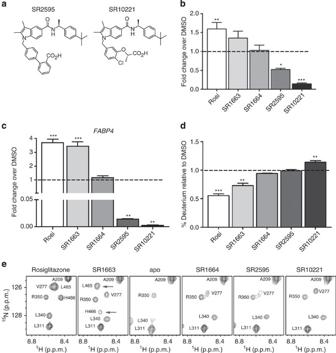Figure 2: Structure guided design of PPARγ inverse agonists. (a) Chemical structures of SR2595 and SR10221. (b) Transcriptional activity of a PPARγ:PPRE-Luciferase promoter–reporter assay in 1 μM treated HEK293T cells (n=3). (c) Quantitative PCR analysis of mRNA extracts from 1 μM treated, differentiated 3T3-L1 adipocytes for adipogenic markerFABP4(n=3). (d) HDX of PPARγ helix 12 peptide SLHPLLQEIYKDLY (PPARγ1 residues 492–505) after 30-s D20 incubation in the presence of ligand relative to DMSO control (n=3). (e) Two-dimensional [1H,15N]-TROSY-HSQC NMR data for PPARγ LBD in the presence of the indicated ligands; arrows indicate resonances near helix 12 that are stabilized by rosiglitazone and SR1663 only. Error bars, s.e.m; one-way analysis of variance, Dunnett’spost hoctest *P<0.05, **P<0.01, ***P<0.001. Figure 2: Structure guided design of PPARγ inverse agonists. ( a ) Chemical structures of SR2595 and SR10221. ( b ) Transcriptional activity of a PPARγ:PPRE-Luciferase promoter–reporter assay in 1 μM treated HEK293T cells ( n =3). ( c ) Quantitative PCR analysis of mRNA extracts from 1 μM treated, differentiated 3T3-L1 adipocytes for adipogenic marker FABP4 ( n =3). ( d ) HDX of PPARγ helix 12 peptide SLHPLLQEIYKDLY (PPARγ1 residues 492–505) after 30-s D 2 0 incubation in the presence of ligand relative to DMSO control ( n =3). ( e ) Two-dimensional [ 1 H, 15 N]-TROSY-HSQC NMR data for PPARγ LBD in the presence of the indicated ligands; arrows indicate resonances near helix 12 that are stabilized by rosiglitazone and SR1663 only. Error bars, s.e.m; one-way analysis of variance, Dunnett’s post hoc test * P <0.05, ** P <0.01, *** P <0.001. Full size image Pharmacological repression of PPARγ promotes osteogenesis As PPARγ deficiency in transgenic mouse models results in enhanced bone formation [7] , pharmacological repression of the receptor emerges as a therapeutic strategy to phenocopy these desirable osteogenic effects. Treatment of cultured human MSCs with SR2595 induced a statistically significant increase in osteogenic differentiation as measured by calcium phosphatase deposition ( Fig. 3a ). This was accompanied by increased expression of bone morphogenetic proteins BMP2 and BMP6 ( Fig. 3b ). Similar effects were observed with short interfering RNA-mediated PPARγ silencing in human MSCs ( Fig. 3c,d ), and together demonstrate that pharmacological PPARγ repression can induce MSC differentiation towards the osteogenic lineage. 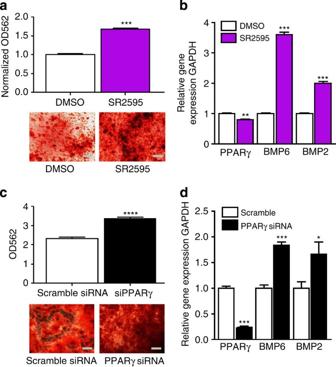Figure 3: Pharmacological repression of PPARγ promotes osteogenesis. (a) Alizarin red staining and quantification of MSCs treated with 1 μM SR2595 (n=3); scale bar, 1 mm. (b) Quantitative PCR (qPCR) analysis of mRNA extracts from 1 μM SR2595 treated MSCs (n=3). (c) Alizarin red staining and quantification of MSCs treated with PPARγ short interfering RNA (siRNA;n=3); scale bar, 1 mm. (d) qPCR analysis of mRNA extracts from siRNA treated MSCs (n=3). Error bars, s.e.m; one-way analysis of variance, Dunnett’spost hoctest *P<0.05, **P<0.01, ***P<0.001, ****P<0.0001. Figure 3: Pharmacological repression of PPARγ promotes osteogenesis. ( a ) Alizarin red staining and quantification of MSCs treated with 1 μM SR2595 ( n =3); scale bar, 1 mm. ( b ) Quantitative PCR (qPCR) analysis of mRNA extracts from 1 μM SR2595 treated MSCs ( n =3). ( c ) Alizarin red staining and quantification of MSCs treated with PPARγ short interfering RNA (siRNA; n =3); scale bar, 1 mm. ( d ) qPCR analysis of mRNA extracts from siRNA treated MSCs ( n =3). Error bars, s.e.m; one-way analysis of variance, Dunnett’s post hoc test * P <0.05, ** P <0.01, *** P <0.001, **** P <0.0001. Full size image Effect of PPARγ repression on metabolic parameters The primary concern with the development of repressive PPARγ inverse agonists is whether they will have negative consequences on metabolic parameters, as the TZD class of insulin sensitizers are potent full agonists. These concerns are partly allayed by the findings that insulin-sensitizing efficacy can be decoupled from PPARγ activation [10] , along with transgenic PPARγ haploinsufficiency resulting in favourable metabolic outcomes [11] , [12] . To determine whether pharmacological PPARγ repression would impair insulin sensitivity, SR2595 was administered chronically to lean C57BL/6J mice for 21 days. The pharmacokinetic properties of SR2595 were sufficient to support once daily oral dosing at 20 mg kg −1 ( Supplementary Fig. 2a,b , plasma exposure and drug concentration in epidiymal white adipose tissue (WAT), respectively). Lean C57BL/6J mice treated with SR2595 demonstrated no significant change in insulin sensitivity as determined by insulin tolerance test ( Supplementary Fig. 3a ), nor fasting insulin levels ( Supplementary Fig. 3b ). In addition, no change in food consumption or body weight was observed during the treatment period ( Supplementary Fig. 3c,d ). In summary, we have identified the structural mechanism by which SR1664 actively antagonizes PPARγ, and extended this work to design the inverse agonist SR2595. Similar SAR was first reported with the oestrogen receptor antagonist tamoxifen [13] , suggesting a broadly applicable strategy for altering the pharmacology of additional SPPARγM scaffolds [14] , [15] . Further broadening the applicability of these findings is the observation that PPARγ F282 is evolutionarily conserved in several nuclear receptors that form obligate RXRα heterodimers including PPARα, PPARδ, LXRα, LXRβ and FXR [16] . Applying this SAR to identify natural antagonists and based on the crystal structures of PPARγ in complex with endogenous fatty acids [17] , we would predict that esterification of fatty acids with a bulky substituent would mimic the steric clash observed with SR1664. Cyclic phosphatidic acid, a putative endogenous PPARγ antagonist fits this profile [18] , further implicating the enzymatic pathways regulating endogenous negative regulators of PPARγ as critical for maintaining metabolic and bone homeostasis. The therapeutic utility of pharmacological PPARγ repression is further suggested by several studies that apply genetic receptor ablation or covalent PPARγ antagonists GW9662 and T0070907 that demonstrate efficacy in cancer [19] , [20] , [21] , obesity [22] , [23] , [24] , arterial neointima formation [25] and bone formation [26] . SR2595 has sufficient pharmacokinetic properties to support animal studies, and the closely matched pharmacokinetics of the biaryl indole series described here provides a useful system to probe PPARγ transcriptional activity in vivo . SR2595 (S)-4′-((5-((1-(4-( tert -butyl)phenyl)ethyl)carbamoyl)-2,3-dimethyl-1H-indol-1-yl)methyl)-[1,1′-biphenyl]-2-carboxylic acid. Commercially available ethyl 2,3-dimethyl-1 H -indole-5-carboxylate was N -alkylated with commercially available tert -butyl 4′-(bromomethyl)biphenyl-2-carboxylate using NaH in DMF. The corresponding ethyl ester was hydrolysed using aqueous NaOH in ethanol to give the acid, which was coupled with (S)-1-(4-( tert -butyl)phenyl)ethan-1-amine hydrochloride (synthesis already described in patent) using 2-(3 H -[1,2,3]triazolo[4,5–b]pyridin-3-yl)-1,1,3,3-tetramethylisouronium hexafluorophosphate(V) (HATU) and diisopropylethylamine in CH 2 Cl 2 to give the amide. Final deprotection of the tert -butyl ester using 30% trifluoroacetic acid in CH 2 Cl 2 and purification by flash chromatography (ethyl acetate/hexanes 10–100%) afforded SR2595. Electrospray ionization coupled with mass spectrometry (ESI-MS; m / z ): 548 [M+H] + ; 1 H NMR (400 MHz, dimethylsulphoxide (DMSO)-d 6 ): δ (p.p.m.) 8.59 (d, J= 8.0 Hz, 1H), 8.10 (d, J= 1.5 Hz, 1H), 8.68 (dd, J= 1.0, 7.6 Hz, 1H), 7.63 (dd, J= 1.5, 8.5 Hz, 1H ), 7.51 (dt, J= 1.5, 7.6 Hz, 1H), 7.44 (d, J= 8.8 Hz, 1H), 7.40 (dd, J= 1.2, 7.6 Hz, 1H), 7.31–7.33 (m, 4H), 7.23 (d, J= 8.3 Hz, 2H), 6.98 (d, J= 8.3 Hz, 2H), 5.47 (s, 2H), 5.33 (quint, J= 7.2 Hz, 1H), 2.32 (s, 3H), 2.28 (s, 3H), 1.26 (s, 9H); 13 C NMR (400 MHz, DMSO-d 6 ): δ (p.p.m.) 169.5, 166.5, 148.7, 142.3, 140.4, 139.2, 137.6, 137.3, 134.0, 132.1, 130.8, 130.4, 129.0, 128.5, 127.5, 127.2, 125.9, 125.8, 125.1, 124.8, 120.3, 117.6, 108.7, 107.2, 47.9, 45.6, 40.1, 34.1, 31.1, 22.1, 10.0, 8.8. SR10221 (S)-2-(5-((5-(((S)-1-(4-( tert -butyl)phenyl)ethyl)carbamoyl)-2,3-dimethyl-1H-indol-1-yl)methyl)-2-chlorophenoxy)propanoic acid. Commercially available 2-chloro-5-methylphenol and methyl-D(+)-lactate gave the methyl (S)-2-(2-chloro-5-methylphenoxy)propanoate by a Mitsunobu reaction, follows by the bromination with N-bromosuccinimide and azobisobutyronitrile in CCl 4 . The corresponding compound was N -alkylated with allyl 2,3-dimethyl-1 H -indole-5-carboxylate using NaH in dimethylformamide (DMF). The deprotection of the allyl group by tetrakis(triphenylphosphine)palladium(0) gave the acid, which was coupled with (S)-1-(4-( tert -butyl)phenyl)ethan-1-amine hydrochloride (synthesis already described in patent) using 2-(3 H -[1,2,3]triazolo[4,5–b]pyridin-3-yl)-1,1,3,3-tetramethylisouronium hexafluorophosphate(V) (HATU) and diisopropylethylamine in CH 2 Cl 2 to give the amide. Final hydrolyse of the methyl ester using aqueous LiOH in tetrahydrofuran (THF) and purification by flash chromatography (ethyl acetate/hexanes 10–100%) afforded SR10221. Electrospray ionization coupled with mass spectrometry (ESI-MS; m / z ): 562 [M+H] + ; 1 H NMR (400 MHz, DMSO-d 6 ): δ (p.p.m.) 8.57 (d, J= 8.1 Hz, 1H), 8.08 (d, J= 1.5 Hz, 1H), 7.60 (dd, J= 1.8, 8.6 Hz, 1H), 7.36 (d, J= 8.6 Hz, 1H ), 7.33 (m, 3H), 7.29 (d, J= 8.1 Hz, 1H), 6.79 (d, J= 1.8 Hz, 1H), 6.34 (dd, J= 1.8, 8.1 Hz, 1H), 5.47 (s, 2H), 5.17 (quint, J= 7.1 Hz, 1H), 4.78 (quint, J= 6.8 Hz, 1H), 2.27 (s, 3H), 2.26 (s, 3H), 1.50 (d, J= 6.8 Hz, 3H), 1.47 (d, J= 7.1 Hz, 3H), 1.26 (s, 9H); 13 C NMR (400 MHz, DMSO-d 6 ): δ (p.p.m.) 172.3, 166.4, 152.9, 148.7, 142.3, 138.8, 137.4, 133.8, 130.8, 127.5, 125.8, 125.2, 124.8, 120.4, 120.1, 119.3, 117.6, 112.4, 108.5, 107.3, 72.5, 47.9, 45.5, 40.1, 34.1, 31.1, 22.2, 18.1, 9.9, 8.7. PPARγ-binding assay PPARγ competitive-binding assay (Invitrogen) was performed according to the manufacturer’s protocol. A mixture of 5 nM glutathione S -transferase fused with the PPARγ ligand-binding domain (GST–PPARγ–LBD), 5 nM Tb-GST-antibody, 5 nM Fluormone Pan-PPAR Green and serial dilutions of compound beginning at 10 μM downwards was added to wells of black 384-well low-volume plates (Greiner) to a total volume of 18 μl. All dilutions were made in Time-resolved (TR)-fluorescence resonance energy transfer (FRET) PPAR assay buffer. DMSO at 2% final concentration was used as a no-ligand control. Experiments were performed in triplicate and incubated for 2 h in the dark before analysis in Perkin Elmer ViewLux ultra HTS microplate reader. The FRET signal was measured by excitation at 340 nm and emission at 520 nm for fluorescein and 490 nm for terbium. The fold change over DMSO was calculated by 520 nm/490 nm ratio. Graphs were plotted in GraphPad Prism as fold change of FRET signal for each compound over DMSO-only control and effector concentration for half-maximum response calculated. Cell-based transactivation assay HEK293T cells (ATCC; cat# CRL-3216) were co-transfected in batch by adding 4.5 μg full-length human PPARγ2-pCMV-AN-DDK or full-length human mutant PPARγ2-F282A-pCMV-AN-DDK, with 4.5 μg 3 × multimerized PPRE-luciferase reporter and 27 μl X-treme Gene 9 transfection reagent in serum-free Opti-MEM reduced serum media (Gibco). After 18-h incubation at 37 °C in a 5% CO 2 incubator, transfected cells were plated in quadruplicate in white 384-well plates (Perkin Elmer) at a density of 10,000 cells per well. After replating, cells were treated with either DMSO only or the indicated compounds in increasing doses from 2 pM to 10 μM. After 18-h incubation, treated cells were developed with Brite Lite Plus (Perkin Elmer) and read in 384-well Luminescence Perkin Elmer EnVision Multilabel plate reader. Graphs were plotted as fold change of treated cells over DMSO-treated control cells. Crystallography The PPARγ LBD was purified as previously reported using an N-terminal 6 × polyhistidine tag [8] . Purified protein was concentrated to 10 mg ml −1 and stored in 20 mM Tris 8.0, 10 mM NaCl and 1 mM TCEP. The SR1664 ligand bound structure was produced by co-crystallization and the SR1663 structure was produced by soaking apo PPARγ LBD T447F crystals with 10 mM compound for 7 days. SR1664 was incubated with PPARγ LBD in a 10:1 (ligand:protein) ratio and the complex was isolated using a fast protein liquid chromatography (FPLC) size exclusion column (Superdex 200, GE Health Sciences). Crystals of the SR1664–LBD complex were formed using a hanging drop vapour diffusion method; crystals formed within 1 week were cubic in morphology, and grew to ∼ 150 μm in each dimension. Crystals were formed at 298 K using 1 μl of well solution, 1 μl of protein complex and 500 μl of well solution. The well solution consisted of 2 M ammonium sulfate. Apo crystals of the PPARγ LBD were also grown by the vapour diffusion method at 298 K and a hanging drop. Apo crystals were formed with 1 μl of well solution, 1 μl of protein complex and 500 μl of well solution; the well solution consisted of 1 M sodium citrate and 0.1 M HEPES 8.0. Apo crystals formed within 3 weeks were cubic in morphology, and grew to ∼ 300microns in each dimension. Apo crystals were soaked with SR1663 for 2 weeks at a final concentration of 1 mM in the drop. Both SR1664 co-crystals and SR1663 soaked crystals were transferred to well solutions containing 15% ethylene glycol for use as a cryo-protectant. All data collection were performed with synchrotron radiation at SSRL beamline 11-1 at 100 K. The 0.2 o oscillations with 1.2 s exposures were collected for a total of 240° at a wavelength of 1.03 Å. Data processing were carried out using HKL2000 (ref. 27 ). Both crystals were of space group C2 consistent with previously published PPARγ LBD crystal structures. Data processing and refinement parameters can be found in Table 1 . The phase problem was overcome by means of molecular replacement using PDB:2Q59 (stripped of water molecules and ligands) as a search model [8] . Refinement was carried out using iterative rounds of refinement using phenix.refine followed by manual rebuilding in Coot [28] until R-factors converged. Molprobity was used for structure validation. Kicked 2F0-FC electron density maps were calculated for both ligands ( Supplementary Fig 4 ). The SR1664 crystal structure had 96.8% residues in favoured Ramachandran positions. Both structures were deposited in the protein data bank: SR1664 as PDB:4R2U and SR1663 as PDB:4R65. HDX coupled with mass spectrometry Solution-phase amide HDX experiments were carried out using a fully automated system as described previously [29] . Ten micromolar of HIS-PPARγ LBD protein (20 mM KPO4 pH 7.4, 50 mM KCl) was preincubated with 1:2 M excess of compound. Five microlitre of protein solution was mixed with 20 μl of D 2 O-containing HDX buffer (20 mM KPO4 pH 7.4, 50 mM KCl) and incubated at 4 °C for 10, 30, 60, 900 and 3,600 s. Following on-exchange, unwanted forward or back exchange was minimized and the protein was denatured by dilution with 25 ul of quench solution (0.1% v/v trifluoroacetic acid (TFA) in 3 M urea). Samples were then passed through an immobilized pepsin column (prepared in house [30] ) at 200 μl min −1 (0.1% v/v TFA, 15 °C) and the resulting peptides were trapped on a C 8 trap column (Hypersil Gold, Thermo Fisher). The bound peptides were then gradient eluted (5-50% CH 3 CN w/v and 0.3% w/v formic acid) across a 2 × 50 mm C 18 high-performance liquid chromatography column (Hypersil Gold, Thermo Fisher) for 5 min at 4 °C. The eluted peptides were then subjected to electrospray ionization directly coupled with a high-resolution Orbitrap mass spectrometer (Exactive, Thermo Fisher). Each HDX experiment was carried out in triplicate and the intensity weighted average m / z value (centroid) of each peptide isotopic envelope was calculated with in-house HDX Workbench software [31] ( Supplementary Fig. 5 ). NMR spectroscopy 15 N PPARγ LBD protein was expressed and purified as described previously [32] , with a final NMR buffer of 20 mM KPO 4 (pH 7.0 or 7.4) 50 mM KCl, 0.5 mM EDTA. To prepare liganded samples, 8 μM protein was loaded ∼ 1:1 with ligand dissolved in DMSO-d 6 and concentrated to 300 μM, followed by addition of 10% D 2 O and 0.05% sodium azide. Two-dimensional [ 1 H, 15 N]-transverse relaxation optimized spectroscopy (TROSY)-heteronuclear single quantum coherence (HSQC) experiments were performed on a 700 MHz ( 1 H frequency) Bruker instrument at a calibrated temperature of 298 K. Data were processed using Topspin 3.0 (Bruker) and analysed using NMRViewJ (One Moon Scientific). NCoR peptide recruitment assay Tb-α-HIS (7.5 nM; Invitrogen) and 10 μM of ligand were incubated in complete TR-FRET PPAR assay buffer (Invitrogen) containing 7.5 nM PPARγ protein (Invitrogen) or 7.5 nM mutated PPARγ F282A. After 1-h incubation at room temperature, 30 μM NCoR NR box 2-1 peptide (THRLITLADHICQIITQDFAR; LifeTein) was added and incubated for an additional 4 h at room temperature, kept in the dark. The FRET signal was measured by excitation at 340 nm and emission at 520 nm for fluorescein and 490 nm for terbium in Perkin Elmer ViewLux ultra HTS microplate reader. The fold change over DMSO was calculated by 520 nm/490 nm ratio. Graphs were plotted in GraphPad Prism as fold change of FRET signal for each compound over DMSO-only control. 3T3-L1 adipogenesis assays 3T3-L1 cells (ATCC; cat# CL-173) were seeded at 50,000 cells per ml in 12-well dish (Corning) with 1 × DMEM (CellGro) containing 10% foetal bovine serum (FBS; GIBCO) and incubated overnight at 37 °C, 5% CO 2 . The following day, cells were treated with 1 μM compound and MDI cocktail consisting of 0.5 mM 3-iso-butyl-1-methylxanthine, 1 μM dexamethasone and 5 μg ml −1 insulin. Following 2-days of incubation, cells were treated with 1 μM fresh compound diluted in 1 × DMEM+10% FBS. After incubating for 6 days, cells were stained with oil red or harvested and lysed. RNA was extracted using RNeasy Mini Kit (Qiagen). Subsequently, complementary DNA was generated using High Capacity Reverse Transcription Kit (Applied Biosystems). Expression levels of PPAR-related genes were measured using Applied Biosystems 7500 Real-Time PCR system. Relative gene expression was calculated and plotted using GraphPad Prism Software. Osteogenic differentiation of mesenchymal stem cells MSCs were harvested from small volume aspirates of the iliac crest from healthy adult volunteers by the Center for Preparation and Distribution of Adult Stem Cells formerly at Tulane University School of Medicine (New Orleans, LA, USA) and currently at Texas A&M Health Science Center (Temple, TX, USA). Mononuclear cells were recovered from a ficoll (Ficoll-Plaque, Pharmacia; Peapack, NJ, USA) gradient, washed using Hank’s balanced salt solution and centrifuged at 500 g for 10 min. Mononuclear cells were then plated at 5,000 cells per cm 2 and cultured in complete culture medium consisting of alpha-minimum essential medium supplemented with 2 mM L -glutamine, 17% FBS (HyClone, Logan, UT, USA, http://www.hyclone.com ) 100 U ml −1 of penicillin, and 100 μg ml -1 of streptomycin at 37 °C in a humidified incubator with 5% CO 2 . After 24 h, the non-adherent cells were removed and adherent cells were cultured to 70% confluence with media changes every 2–3 days. Cells were then harvested using 0.2% trypsin-EDTA and secondary cultures were routinely plated at 500–1,000 cells per cm 2 and expanded as described above. Osteogenic differentiation was performed by culturing MSCs in osteogenic induction media (DMEM low glucose supplemented with 10% foetal bovine serum, 10 mM β-glycerophosphate, 50 μg ml −1 L -ascorbic acid 2-phosphate1% penicillin/streptomycin) containing vehicle or compounds for 15 days with media changes every 2–3 days. In experiments involving PPARγ knockdown, osteogenic induction media was added 24 h after short interfering RNA (10 nM) transfection. After 15 days of differentiation, cells were washed with PBS, incubated in 10% neutral buffered formalin for 1 h at room temperature, washed with deionized water and stained with Alizarin Red S for 20 min at room temperature. Monolayers were then rinsed 3 × with deionized water until clear, washed with PBS, stain was then extracted with 10% (w/v) cetylpyridinium chloride in 10 mM sodium phosphate, pH 7.0 for 15 min at room temperature and the amount of extracted dye quantified spectroscopically at 562 nm. Spectroscopic analysis performed using a SpectraMax M5e Multi-Mode Microplate Reader (Molecular Devices, LLC.) and images acquired using a Leica DMI3000B upright fluorescent microscope attached to a DFC295 digital camera (Micro Optics of Florida,Inc., Davie, FL, USA, http://www.microopticsfl.com ). RNA was isolated from cell monolayer after 5 days of differentiation for gene expression studies. Gene expression analysis Total RNA was isolated from cells or tissues using TRIzol reagent (Invitrogen). The RNA was reverse transcribed using the ABI reverse transcription kit. Quantitative PCR reactions were performed with SYBR green fluorescent dye using an ABI9300 PCR machine. Relative messenger RNA expression was determined by the ΔΔ- C t method normalized to GAPDH or TATA box binding protein (TBP) levels. The sequences of primers used in this study are found in Supplementary Table 2 . Animals All animal experiments were performed according to procedures approved by Scripps Florida IACUC Committee. Male C57BL/6J mice were purchased from the Jackson Laboratory (7-week-old) and fed a regular chow diet through experiments. The mice were dosed by oral gavage once daily with 5 mg kg −1 rosiglitazone or 20 mg kg −1 SR2595 for 21 days. For insulin tolerance tests, mice were fasted overnight before intraperitoneal injection of 0.75 U kg −1 insulin (Sigma). Glucose was then measured by tail vein bleeds at the indicated intervals using an OneTouch Ultra2 glucometer. Plasma insulin concentration was determined by enzyme-linked immunosorbent assay (Millipore mouse/rat insulin. cat # EZRMI-13 K). Accession codes: Coordinates and structure factors have been deposited in the Protein Data Bank (PDB) with accession codes 4R2U (for SR1664) and 4R65 (for SR1663). How to cite this article: Marciano, D.P. et al . Pharmacological repression of PPARγ promotes osteogenesis. Nat. Commun. 6:7443 doi: 10.1038/ncomms8443 (2015).